Promotion of oxygen reduction by a bio-inspired tethered iron phthalocyanine carbon nanotube-based catalyst Electrocatalysts for oxygen reduction are a critical component that may dramatically enhance the performance of fuel cells and metal-air batteries, which may provide the power for future electric vehicles. Here we report a novel bio-inspired composite electrocatalyst, iron phthalocyanine with an axial ligand anchored on single-walled carbon nanotubes, demonstrating higher electrocatalytic activity for oxygen reduction than the state-of-the-art Pt/C catalyst as well as exceptional durability during cycling in alkaline media. Theoretical calculations suggest that the rehybridization of Fe 3d orbitals with the ligand orbitals coordinated from the axial direction results in a significant change in electronic and geometric structure, which greatly increases the rate of oxygen reduction reaction. Our results demonstrate a new strategy to rationally design inexpensive and durable electrochemical oxygen reduction catalysts for metal-air batteries and fuel cells. Polarization due to the oxygen reduction reaction (ORR) still contributes significantly to the energy efficiency of several fuel cells and metal-air batteries [1] , [2] , because of the exceptionally high O=O bond energy (498 kJ mol −1 ) and the sluggish nature of ORR. Although Pt and its alloys are known as the most efficient catalysts for activation of the strong oxygen–oxygen double bond [3] , [4] , [5] , their application is limited by high costs and scarce reserves. To overcome this problem, low-cost, non-precious metal catalysts have attracted much attention in the search for an alternative catalyst for a new generation of fuel cells and metal-air batteries [6] , [7] , [8] , [9] , [10] , [11] , [12] . Among the non-precious catalysts studied, Fe–N–C catalysts have attracted the most interest owing to their low-cost and facile preparation methods [13] , [14] . However, today’s Fe–N–C catalysts still suffer from low activity and poor durability, especially for unpyrolysed Fe–N–C catalysts. The typical cycle life for unpyrolysed Fe–N–C catalysts is less 100 cycles in either acidic or basic media [15] , [16] . It is a great challenge to replace Pt-based catalysts by inexpensive Fe–N–C catalysts while maintaining similar performance in practical applications. Metal macrocycles, such as metal (iron or cobalt) porphyrins and phthalocyanines, are the precursors most widely used to prepare the ORR catalysts. Metal macrocycles were first observed to facilitate ORR in fuel cells in 1964 (ref. 17 ), and were then thoroughly investigated as potential cathode catalyst in fuel cells and metal-air batteries [18] . To date, however, limited progress has been made in improving their electrocatalytic activity and durability [19] . In particular, macrocycle compounds have been demonstrated for a long time to suffer from severe degradation in fuel cell environments due to demetalation and/or degradation of iron phthalocyanine (FePc) by ORR intermediates [20] , [21] . Traditional strategy to enhance the activity and durability of the Fe–N–C type of non-precious metal catalysts involves high temperature pyrolysis process, which resulted in complicated chemical and electronic structure of metal ions [22] , [23] , [24] . Although the pyrolysed catalysts offer better performance toward ORR than those without pyrolysis, their chemical structures undergo a complicated and unpredictable transformation during the heat-treatment [25] . Accordingly, the nature of the active sites in heat-treated Fe–N–C catalyst is still unclear [26] , [27] . The unpredictable structural change and unclear catalytic mechanism make it difficult to achieve rational design of Fe–N–C catalyst for ORR. Alongside the pyrolysis strategy, state-of-the-art synthetic techniques have been used to modify the geometric and electronic structure of metal macrocycles and its derivatives to improve its performance toward ORR [16] , [28] , [29] . However, most of the synthetic strategies focus on four-coordinated systems in an effort to change the accommodating space for oxygen molecules between cofacial porphyrins in its dyads and little attention has been paid to tuning the coordination environment of the Fe ion [30] , [31] . By tuning the steric and electronic structure of catalysts, a rationally designed, synthetic Fe–N–C system should offer a more positive half-wave potential, and greater durability by modifications with proper functional groups [16] . To date, however, all reported synthesized Fe–N–C catalysts are still inadequate for practical applications because of limited durability and low activity. In nature, on the other hand, the billion-year-old ORR catalyst cytochrome c oxidase located in respiratory chain also contains an active site of iron(II)-porphyrin structure [32] . Unlike the synthetic metal macrocycle catalysts for ORR, however, the iron centre in biological systems contains five-coordinated structure with an axial ligand from the back side. Inspired by this unique feature of the active site in cytochrome c oxidase, we design a new class of ORR catalyst using pyridine-functionalized carbon nanotubes (CNTs) to anchor FePc molecules and provide the axial ligand for the iron centre. At the same time, the CNTs provide an easy pathway for fast electron transfer from the current collector to the ORR active sites. Preparation of FePc–Py–CNTs catalyst We synthesized the composite of FePc and single-walled CNTs (FePc–Py–CNTs) from covalent functionalization of single-walled CNTs (Py–CNTs) ( Supplementary Fig. S1 ). In this approach, pyridyl groups (Py) were first anchored on the walls of CNTs, taking advantage of the diazonium reaction. FePc was then coordinated to Py–CNTs through the bond formed between nitrogen atom in pyridine and iron centre in FePc ( Fig. 1a ). The reasons that we choose pyridine as linkers are as follows: (1) pyridine can be easily anchored on the walls of CNTs through covalent bond; (2) the coordination bond between pyridine and FePc is strong, forming a stable structure of FePc–Py–CNTs composite; (3) pyridine contains aromatic structure and has small molecule size, which favors fast electron transfer from CNTs to FePc for ORR; and (4) pyridine as the axial ligand changes the coordination number of iron centre, resulting in an electronic and geometrical structure of iron ion for efficient ORR. To prove that FePc was covalently anchored on CNTs, several characterization techniques were used to investigate the physical and chemical structure of this FePc–Py–CNTs composite. 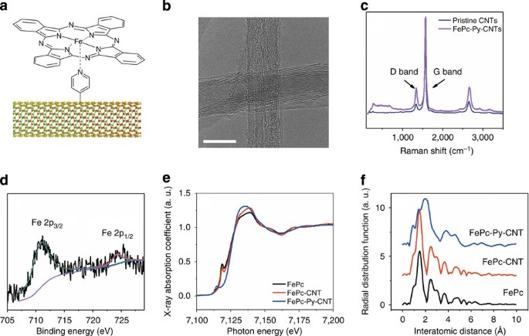Figure 1: Schematic view and characterization of catalysts. (a) Schematic diagram of the structure of FePc–Py–CNTs composite. (b) HR-TEM imgage of FePc–Py–CNTs composite. Scale bar, 10 nm. (c) Raman spectra of pristine CNTs and FePc–Py–CNTs composite. D-band and G-band peaks are marked with arrows. (d) XPS Fe2pspectra of FePc–Py–CNTs composite. (e) X-ray absorption near edge structure (XANES) spectra of FePc, FePc–CNTs and FePc–Py–CNTs. (f) Fourier-transformed module of EXAFS signals for FePc, FePc–CNTs and FePc–Py–CNTs. Figure 1: Schematic view and characterization of catalysts. ( a ) Schematic diagram of the structure of FePc–Py–CNTs composite. ( b ) HR-TEM imgage of FePc–Py–CNTs composite. Scale bar, 10 nm. ( c ) Raman spectra of pristine CNTs and FePc–Py–CNTs composite. D-band and G-band peaks are marked with arrows. ( d ) XPS Fe 2p spectra of FePc–Py–CNTs composite. ( e ) X-ray absorption near edge structure (XANES) spectra of FePc, FePc–CNTs and FePc–Py–CNTs. ( f ) Fourier-transformed module of EXAFS signals for FePc, FePc–CNTs and FePc–Py–CNTs. Full size image Characterization of FePc–Py–CNTs catalyst Thermalgravimetric analysis of Py–CNTs and FePc–Py–CNTs indicated that the functionalization reactions were successful ( Supplementary Fig. S2 ) and the stoichiometry (nanotube carbons bearing pyridine moiety, Py/C) is ~1/48, which is slightly lower than the results reported in a previous study [33] . The Fe content in FePc–Py–CNTs was confirmed to be 2.56 wt% by ICP-AES. The D-band intensity of the FePc–Py–CNTs composite was higher than that of pristine SWCNTs ( Fig. 1c ), another indication of covalent functionalization of CNTs. The high-resolution transmission electron microscope (HR-TEM) image in Fig. 1b shows representative structure of the FePc–Py–CNTs composite. After functionalization, surface bumps were found along the sidewalls of CNTs, which are revealed as covalently functionalized moieties attached to CNTs [33] . Images of low magnification TEM and scanning electron microscope show individual and bundle of CNTs ( Supplementary Fig. S3 ). The X-ray photoelectron spectroscopy (XPS) and extended X-ray absorption fine structure (EXAFS) were used to investigate the electronic structure of iron ion in FePc–Py–CNTs composite. The XPS Fe 2p core level spectra show the peak position at 711.1 eV for the FePc–Py–CNTs composite ( Fig. 1d ). On the other hand, the Fe 2 p 3/2 core level spectra in a physical mixture of FePc and SWCNTs (labelled as FePc–CNTs) was down shifted to 709.9 eV ( Supplementary Fig. S4 ). As Fe ion is coordinated with the Py group at the axial direction in FePc–Py–CNTs, the extra ligand leads to the change of electron density on Fe, resulting in more positive iron ion than FePc–CNTs. As a result, the peak position of Fe 2p shifted to higher binding energy. The XPS N 1s peak of FePc–Py–CNTs was shown at 398.5 eV ( Supplementary Fig. S5 ). It is worth noting that no peaks of N 1s and Fe 2p for pristine CNTs were observed in the spectra ( Supplementary Fig. S6 ). To further understand the electronic structure of Fe in catalysts, which is critically important for ORR activity, we carried out EXAFS measurements. Figure 1e shows the X-ray absorption Fe K-edge spectra of FePc and its composites. Different edge structure is observed with respect to photon energy for FePc–Py–CNTs composite, while pristine FePc and FePc–CNTs remain similar edge structure shape. A clear shift toward the higher energy region is observed for FePc–Py–CNTs in comparison with pristine FePc and FePc–CNTs, indicating a higher oxidation state of iron ion in FePc–Py–CNTs. This is consistent with the XPS results. In addition, the shoulder peak relates to an electric-dipole allowed transition of 1s electron to 4p z orbital followed by ligand-to-metal charge transfer process. The shoulder peaks featured at ~7118.4 eV for FePc and FePc–CNTs is typical characteristics of square-planar D 4 h local symmetry of Fe ion surrounded by four-coordinated nitrogen ligands. For FePc–Py–CNTs, the distinct shoulder peak is located at ~7114.7 eV, suggesting an effective change of local symmetry from square-planar to five-coordination system by additional binding of axial ligands. It is also seen that the radial distribution around iron ion is very different ( Fig. 1f ). In the EXAFS spectra, unlike the FePc and FePc–CNTs with only four-coordinated nitrogen in the equatorial direction under D 4 h symmetry, the additional Fourier-transformed peak of FePc–Py–CNTs around 2 Å may correspond to the axial-coordinated ligands. Electrochemical evaluation of FePc–Py–CNTs catalyst To investigate the electrocatalytic activity of FePc–Py–CNTs composite for ORR, the as-synthesized composite catalyst was tested in 0.1 M KOH electrolyte solution saturated with O 2 in a standard 3-electrode electrochemical cell. To benchmark the activity of FePc–Py–CNTs composite, a state-of-the-art commercial Pt/C catalyst (20% Pt on Vulcan XC-72, Premetek) was tested under the same conditions. A profound cathodic current for the FePc–Py–CNTs composite is observed in O 2 saturated 0.1 M KOH solution ( Supplementary Fig. S7 ). Surprisingly, the FePc–Py–CNTs exhibit exceptionally high ORR activity, evident from an unprecedentedly positive half-wave potential ( E 1/2 ) at ~0.915 V versus reversible hydrogen electrode (RHE) ( Fig. 2a ). On the other hand, the E 1/2 value of FePc–CNTs and Py–CNTs are much lower than that of FePc–Py–CNTs composite ( Supplementary Fig. S8 ). The promotion of oxygen reduction is attributed to the more positive Fe active centre in the FePc–Py–CNTs composite than that in the FePc–CNTs composite. It should be noted that the state-of-the-art Pt/C catalyst exhibited a E 1/2 value at 0.88 V (versus RHE) ( Fig. 2a ), which is consistent with previously reported results in literatures [6] . The half-wave potential for the FePc–Py–CNTs composite was more positive by ~35 mV than that for the commercial Pt/C catalyst and most of the results previously reported for NMPCs ( Supplementary Table S1 ), indicating that the as-synthesized composite catalyst has very high electrocatalytic activity toward ORR in alkaline media. In addition, it is noted that the ORR activity of FePc–Py–CNTs is also much higher than that of FePc–CNTs in an acid medium (0.5 M H 2 SO 4 eletrolyte), as shown in Supplementary Fig. S9 . 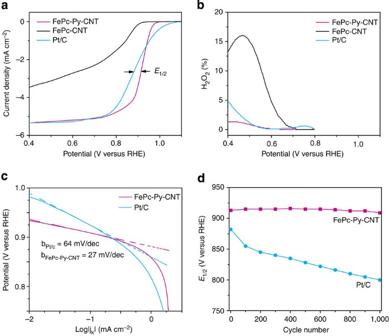Figure 2: Electrochemical evaluation of catalysts. (a) Linear scanning voltammograms of FePc–CNTs, FePc–Py–CNTs and commercial Pt/C catalyst. (b) HO2−yield measured with various catatlys of FePc–CNTs, FePc–Py–CNTs and commercial Pt/C catalyst. (c) Tafel plots of FePc–Py–CNTs and commercial Pt/C catalyst. (d) Half-wave potential as a function of cycle number of FePc–Py–CNTs and commercial Pt/C catalyst during durability test. Electrolyte: 0.1 M KOH, scan rate: 10 mV s−1. Figure 2: Electrochemical evaluation of catalysts. ( a ) Linear scanning voltammograms of FePc–CNTs, FePc–Py–CNTs and commercial Pt/C catalyst. ( b ) HO 2 − yield measured with various catatlys of FePc–CNTs, FePc–Py–CNTs and commercial Pt/C catalyst. ( c ) Tafel plots of FePc–Py–CNTs and commercial Pt/C catalyst. ( d ) Half-wave potential as a function of cycle number of FePc–Py–CNTs and commercial Pt/C catalyst during durability test. Electrolyte: 0.1 M KOH, scan rate: 10 mV s −1 . Full size image To gain deeper insight into the mechanism of ORR, it is necessary to identify the active centre in FePc–Py–CNTs. As shown in Supplementary Fig. S10 , the ORR activity was significantly inhibited by the introduction of KCN, suggesting that the Fe ion is the active centre in the catalyst. This is further confirmed by the observation that the ORR activity was recovered by simply rinsing the electrode with water to remove CN − ions absorbed on the active sites. The yield of peroxide species (HO 2 − ) reflects the mechanism of ORR. In addition, high yield of HO 2 − may damage the stability of catalyst [34] . The HO 2 − yield over FePc–Py–CNTs is below 1.5% at the whole potential range from 0.4–0.8 V ( Fig. 2b ), which is much lower than that for its counterpart of FePc–CNTs. The very high electrocatalytic activity of FePc–Py–CNTs for ORR is also reflected by its low Tafel slop of diffusion-corrected kinetic current density, which is ~27 mV per decade at low overpotential ( Fig. 2c ). As a reference, the Tafel slope of commercial Pt/C is ~64 mV per decade. Such low Tafel slope for FePc–Py–CNTs indicates that the protonation of O 2− on the active sites of catalyst is the rate limiting step [6] , [35] . In addition, it is well known that the number of electrons involved in ORR is another important parameter relevant to the activity of catalysts. The direct four-electron pathway mechanism for ORR is desirable because of its high efficiency and non-corrosion product. The low level of HO 2 − yield with FePc–Py–CNTs composite suggests a four-electron pathway for ORR. The number of electrons for FePc–Py–CNTs was determined to be ~4.05 from Koutecky–Levich’s equation ( Supplementary Fig. S11 ), suggesting that O 2 is reduced on the FePc–Py–CNTs composite most likely through a direct four-electron pathway. The calculated average value of n is ~4.02 for Pt/C catalyst ( Supplementary Fig. S11 ). More importantly, the FePc–Py–CNTs composite catalyst exhibited excellent durability, unlike most unpyrolysed Fe–N–C catalysts and artificial synthetic metal macrocycles that suffer from very poor durability (less than 100 cycles) in an alkaline electrolyte [15] , [16] . To investigate the durability of this catalyst, the FePc–Py–CNTs composite was cycled from 1.13 to 0.33 V (versus RHE) at a scan rate of 10 mV s −1 in 0.1 M KOH solution saturated with O 2 . As shown in Fig. 2d , very little change in half-wave potential (~5 mV) was observed for the FePc–Py–CNTs composite after 1,000 cycles of potential sweeps, while there was ~80 mV loss of half-wave potential for the commercial Pt/C catalyst under the same conditions. Further, the FePc–Py–CNTs composite retained ~92% of the initial current density at 0.9 V versus RHE after 1,000 cycles, comparing with the ~30% retained for the commercial Pt/C catalyst ( Supplementary Fig. S12 ). As the half-wave potential for FePc–CNTs is much lower than FePc–Py–CNT and Pt/C, we investigated the change of limiting current density for FePc–CNT. Only ~75% of limiting current density was remained for FePc–CNTs after only 100 cycles ( Supplementary Fig. S13 ). In addition to the very high activity and excellent durability, the FePc–Py–CNTs composite also exhibits better methanol tolerance than commercial Pt/C catalyst ( Supplementary Fig. S14 ). To demonstrate the practical application of this catalyst, we used the FePc–Py–CNTs composite as cathode catalyst to evaluate its performance in Zn-air batteries under realistic conditions. A best-practiced method was used to prepare the air electrode, which has been tested by cross-laboratory study [36] . We assembled the Zn-air cells to evaluate the performance of FePc–Py–CNTs, FePc–CNTs and a commercial Pt/C catalyst in these cells with 1–6 M KOH electrolytes ( Supplementary Fig. S15 ). Clearly, as shown in Fig. 3 , the cells with the FePc–Py–CNTs composite exhibited the best performance among all cells tested at different current densities in both electrolytes, which is consistent with the electrochemical half-cell test results. The initial discharge voltage for FePc–Py–CNTs in a Zn-air cell (6 M KOH) reached 1.38 V, suggesting that the catalyst performed as a very good catalyst for ORR under practical conditions. After discharging, the cell voltage with FePc–Py–CNTs catalyst can be recovered by ‘recharging’ (refill the zinc powder and KOH electrolyte) the cells. The cell with FePc–Py–CNTs catalyst can be ‘recharged’ several cycles and was operated over 100 h without visible voltage loss, an indication of excellent durability and robustness of this catalyst ( Supplementary Fig. S16 ). In principle, this FePc–Py–CNTs catalyst can be used in similar electrolyte systems for other applications, such as alkaline fuel cells. 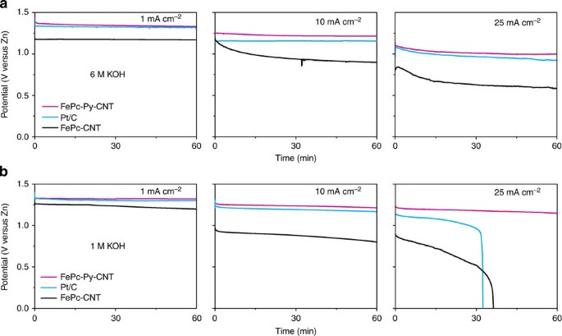Figure 3: Full-cell test of catalysts. Discharge profiles for FePc–Py–CNTs, FePc–CNTs and a commercial Pt/C catalyst at various current densities in Zn-air cells with KOH eletrolytes of different concentrations: (a) 6 M and (b) 1 M. Figure 3: Full-cell test of catalysts. Discharge profiles for FePc–Py–CNTs, FePc–CNTs and a commercial Pt/C catalyst at various current densities in Zn-air cells with KOH eletrolytes of different concentrations: ( a ) 6 M and ( b ) 1 M. Full size image In order to unveil the origin of enhanced catalytic activity and excellent durability of the FePc–Py–CNTs composite catalyst for ORR, spin-polarized density functional theory (DFT)-based calculation was conducted for the four- and five-ligated systems. The adsorption of oxygen molecules, stretching of O–O bond, and the binding energy of OOH ( E ad ) on the active sites are the key parameters which may determine the rate of the ORR process [7] , [37] . As a result of rehybridization of 3 d orbitals with the states of the axial ligand and charge transfer, the geometrical and electronic structure of the five-ligated FePc–Py–CNT system is found to be very different from those of the four-ligated FePc–CNT system. As shown in Fig. 4 , the end-on configurations of O 2 and OOH with stretching of O–O bond (about 8% longer than free O 2 molecule) are observed in both FePc–CNT and FePc–Py–CNT systems. In comparison with FePc-CNT system, higher stretching degree of O–O bond on FePc–Py–CNT system is observed, which makes the dioxygen molecule easier to be broken. The binding energy of O 2 and OOH with FePc–Py–CNT are slightly higher than that of FePc–CNT ( Supplementary Table S2 ), which suggests a favourable adsorption process of O 2 and OOH on the active sites. In addition, a higher charge density near Fermi level in the FePc–Py–CNT system has been found, which may facilitate the ORR process. It is worth noting that the HOO–FePc–Py–CNT system has a lower spin state than the HOO–FePc–CNT system. It has been reported that only specific iron centres in low spin states in pyrolysed Fe–N–C catalysts are responsible for the ORR activity [23] , [27] . 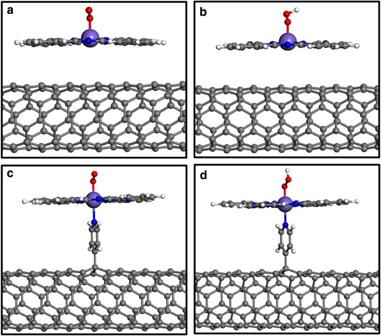Figure 4: Theoretical calculations. (a) Optimized structure of O2adsorbed on FePc–CNT structure. (b) Optimized structure of OOH molecule adsorbed on FePc–CNT structure. (c) Optimized structure of O2adsorbed on FePc–Py–CNT structure. (d) Optimized structure of OOH molecule adsorbed on FePc–Py–CNT structure. The grey, blue, white, red and violet balls represent the carbon, nitrogen, hydrogen, oxygen and iron ion, respectively. Figure 4: Theoretical calculations. ( a ) Optimized structure of O 2 adsorbed on FePc–CNT structure. ( b ) Optimized structure of OOH molecule adsorbed on FePc–CNT structure. ( c ) Optimized structure of O 2 adsorbed on FePc–Py–CNT structure. ( d ) Optimized structure of OOH molecule adsorbed on FePc–Py–CNT structure. The grey, blue, white, red and violet balls represent the carbon, nitrogen, hydrogen, oxygen and iron ion, respectively. Full size image In addition, the displacement of iron ion from the centre of the phthalocyanine ring (R ct-Fe ) due to O 2 adsorption is critical to the stability of the ORR catalyst. Larger displacement of Fe centre corresponds to longer and weaker Fe–N 4 bond ( Supplementary Fig. S17 ), increasing the probability of iron ion dissociation from the aromatic macrocycles, which is commonly believed to be responsible for the degradation in activity [16] . As shown in the optimized structure of FePc–CNT systems ( Fig. 4a ), the iron ion is pulled out of the plane of macrocyclic ring from its original site after adsorption of O 2 and OOH molecule. In contrast, the iron ion remains in the plane of macrocycles in the FePc–Py–CNT system, very close to its original position ( Fig. 4c ). The little displacement of Fe in the FePc–Py–CNT system results in stronger Fe–N bonds than in the FePc–CNT system ( Supplementary Table S2 ), leading to excellent stability. In addition, compared with the four-ligated Fe in the FePc–CNT system, the extra axial coordination bond between Fe and the Py group in the FePc–Py–CNT system is also helpful in reducing the probability of Fe ion dissociation and in enhancing the durability. In conclusion, our bio-inspired FePc–Py–CNTs catalyst has demonstrated exceptionally high durability and electrocatalytic activity for ORR in alkaline media, offering better performance than a commercial Pt/C catalyst. Compared with other unpyrolysed metal macrocycles catalysts, this bio-inspired FePc–Py–CNTs catalyst has achieved much longer cycle life, reaching more than 1,000 cycles in durability test. These results suggest that the FePc–Py–CNTs catalyst is a technologically promising candidate for practical applications in metal-air batteries and alkaline fuel cells. Further, DFT calculations suggest that the origin of the enhanced performance for this bio-inspired catalyst may originate from the electronic structure change of Fe centre in aromatic macrocycle, providing important insight into rational design of metal macrocycles catalysts for other applications such as solar harvesting and catalysts for other redox reactions. Catalyst preparation The synthesis of FePc–Py–CNTs was started from functionalization of CNTs with Py groups using diazonium reaction. Briefly, 4.90 g of NaNO 2 was dissolved in 7 ml H 2 O, and then cooled to 0 °C by ice bath. In all, 6.58 g of 4-aminopyridine (4-AP) was dissolved in 5 ml 4 M HCl, and then cooled to 0 °C by ice bath. The solution of NaNO 2 was added dropwise to 4-AP solution. The resulting yellow solution was maintained at 0 °C in ice bath and stirred for 30 min. Single-walled CNTs ( L -purified Singlewall nanotube, outer diameter <2 nm, 1 g, Lot PS-0607, Catalogue no. 900-1301) was purchased from SES Research (Houston, USA). Before using for synthesis, SWCNTs was purified by being immersed in concentrated HCl solution for 5 days and then refluxed for 5 h, followed by thoroughly washing with water and acetone. The purified SWCNTs was dried overnight at 80 °C in vacuum oven for stock. One hundred milligram of purified SWCNTs was dispersed in 200 ml N , N -dimethylformamide using bath sonicator for 2 h and probe sonicator for 30 min. The SWCNTs solution was cooled to 0 °C by ice bath, and then the yellow solution of NaNO 2 and 4-AP was added dropwise and maintained at 0 °C to prevent the decomposition of diazonium salts. The mixture was reacted at 0 °C for 3 h and then was stirred at room temperature for 15 h. The resulting product (Py–CNTs) was collected by filtering, and then thoroughly washed with 2 M HCl, 2 M NaOH, water and acetone. The Py–CNTs was dried overnight at 80 °C in vacuum oven for stock. Next, the FePc–Py–CNTs composite was prepared by refluxing the mixture of Py-CNTs and FePc in tetrahydrofuran under argon atmosphere. The FePc–CNTs composite was prepared by mixing 100 mg of SWCNTs and 50 mg of FePc. The mixture was shaken in a 5-ml glass vial for 30 min. Then, the mixture was ground in motor for 15 min. Catalyst characterization The material morphology was examined by scanning electron microscope (Nanonova 230, FEI) operating at 10 kV and HR-TEM (JEOL JEM-2100F) operating at 200 kV. XPS analysis was performed using a Thermo Scientific Kα spectrometer (monochromatic Al Kα, 1486.6 eV). Raman spectra was collected on a Micro-Raman system (Alpha 300 s, WITec GmbH) with 532 nm lasers. The thermalgravimetric analysis data were collected under N 2 gas at a heating rate of 5 °C min −1 using a Q600 thermogravimetric analyser (TA Instruments). The Fe content was determined by inductively coupled plasma optical emission spectrometry (ICP-OES, Varian 720-ES). Fe k-edge X-ray absorption spectra, X-ray absorption near edge structure and EXAFS, were collected on BL10C beam line at the Pohang light source-II with a ring current of 100 mA at 3.0 GeV. The monochromatic X-ray beam could be obtained from high-intense X-ray photons of multipole wiggler source using liquid-nitrogen cooled Si (111) double crystal monochromator (Bruker ASC). The X-ray absorption spectroscopic data were recorded for the uniformly dispersed powder samples with a proper thickness on the polyimide film, in transmission mode with N 2 gas-filled ionization chambers as detectors. Higher order harmonic contaminations were eliminated by detuning to reduce the incident X-ray intensity by ~40%. Energy calibration has been simultaneously carried out for each measurement with reference Fe metal foil placed in front of the third ion chamber. The data reductions of the experimental spectra to normalized X-ray absorption near edge structure and Fourier-transformed radial distribution function were performed through the standard XAFS procedure. Catalyst evaluation Rotational ring-disc electrode (RRDE, Ф=4 mm) with glassy carbon was used to evaluate the catalysts. Before use, the electrode was polished to mirror flat with alumina powder. The ink formulation (FePc–Py–CNTs, FePc–CNTs or 20% Pt on Vulcan XC-72, Premeteck) is 10 mg of catalyst, 250 μl of 5 wt% of Nafion in mixture of lower aliphatic alcohols and H 2 O (Sigma-Aldrich) and 1,000 μl of ethanol. The ink was shaken and sonicated in bath sonicator for 1 h. Five microliter of catalyst ink was loaded on the surface of electrode and resulted in a catalyst loading of ~318.5 μg cm −2 . For Pt/C catalyst, the Pt loading is ~63.7 μg Pt cm −2 . Electrochemical test was carried out on IVIUMnSTAT electrochemical analyser by using a typical three-electrode system, with Pt wire as counter electrode and Hg/HgO as reference electrode. The potential difference between Hg/HgO and RHE was measured in H 2 saturated 0.1 M KOH electrolyte and the value is 0.930±0.001 V. The scan rate for all measurements was at 10 mV s −1 from 0.2 to −0.6 V versus Hg/HgO reference electrode. Note that positive scan was recorded for Pt catalyst to remove the side effect of anions adsorption on electrode. In RRDE test, the ring potential was set to 0.4 V versus Hg/HgO reference electrode. Before test, the electrolyte of 0.1 M KOH was saturated with O 2 for at least 30 min, and O 2 purging was kept during electrochemical experiments. The RRDE collection efficiency ( N ) was calibrated in 0.1 M KOH with a 10-mM K 3 Fe(CN) 6 electrolyte. The measured N value is ~0.43 in our system. The H 2 O 2 yield was calculated following the equation: where I r represents the ring current and I d represents the disk current. I r was corrected by subtracting the background current. The number of electrons involved in the reaction was determined from experiment using Koutecky–Levich’s equation: where i , i k , and i d represent measured, kinetic and diffusion-limiting current, respectively, and n is the number of electrons involved in ORR; F is Faraday constant (96,485 C mol −1 ); A is the geometric electrode area (0.1256, cm 2 ); k is the rate constant for oxygen reduction (m s −1 ); C is the saturation concentration of O 2 in 0.1 M KOH solution (1.2 × 10 −6 mol cm −3 ); D is the diffusion coefficient of O 2 in 0.1 m KOH solution (1.9 × 10 −5 cm 2 s −1 ); ν is the kinetic viscosity of solution (0.01 cm 2 s −1 ); and ω is the angular rotation speed (rad s −1 ). In an acid medium, electrochemical tests were performed using a typical three-electrode configuration, with Pt wire as the counter electrode and Ag/AgCl as the reference electrode. The scan rate for all measurements was 10 mV s −1 in a potential range of 0–0.8 V (versus Ag/AgCl reference electrode). Note that positive scan was recorded for Pt catalyst to remove the side effect of anions adsorption on electrode. Before each potential scan, the electrolyte of 0.5 M H 2 SO 4 was saturated with O 2 for at least 30 min, and O 2 purging was kept during electrochemical experiments. KCN poison test was conducted in 0.1 M KOH solution with 10 mM KCN. The scan rate was at 10 mV s −1 from 0.2 to −0.6 V versus Hg/HgO reference electrode. After poison test, the electrode was rinsed with DI water for 30 min to remove KCN. For all the cell tests, zinc powder was used for an anode, and 1 M KOH or 6 M KOH was used for electrolyte. Nylon membrane was used for a separator. The ink formulation (FePc–Py–CNTs, FePc–CNTs or 20% Pt on Vulcan XC-72, Premeteck) is 25 mg of catalyst, 250 μl of 5 wt% of Nafion in mixture of lower aliphatic alcohols and H 2 O (Sigma-Aldrich), and 1,000 μl of ethanol. The ink was shaken and sonicated in bath sonicator for 1 h. The air cathode was prepared by uniformly pasting the catalyst ink on the gas diffusion layer (NARA CELL-TECH). The diameter of an air cathode for full-cell test was 16 mm. The catalyst loading for FePc–Py–CNTs, FePc–CNTs and Pt/C (mass of Pt and C) are same at 600 μg cm −2 . The air cathode was assembled in a home-made zinc-air cell for electrochemical tests. Computational methods Spin-polarized DFT-based calculations are performed using the Vienna ab initio simulation package. Projected augmented wave potentials are used to describe the core electrons. Perdew, Burke and Ernzernhof functional implemented in general gradient approximation was employed to describe the electrons exchange-correlation potential. The Khon-Sham one-electron wave functions are expanded in a plane wave basis set with cutoff energy of 400 eV. The length of CNT and supercell size in the model is enough to render spurious interaction energy between adsorbate and carbon. How to cite this article: Cao, R. et al. Promotion of oxygen reduction by a bio-inspired tethered iron phthalocyanine carbon nanotube-based catalyst. Nat. Commun. 4:2076 doi: 10.1038/ncomms3076 (2013).